Landscape of the mitochondrial Hsp90 metabolome in tumours Reprogramming of tumour cell metabolism contributes to disease progression and resistance to therapy, but how this process is regulated on the molecular level is unclear. Here we report that heat shock protein 90-directed protein folding in mitochondria controls central metabolic networks in tumour cells, including the electron transport chain, citric acid cycle, fatty acid oxidation, amino acid synthesis and cellular redox status. Specifically, mitochondrial heat shock protein 90, but not cytosolic heat shock protein 90, binds and stabilizes the electron transport chain Complex II subunit succinate dehydrogenase-B, maintaining cellular respiration under low-nutrient conditions, and contributing to hypoxia-inducible factor-1α-mediated tumorigenesis in patients carrying succinate dehydrogenase-B mutations. Thus, heat shock protein 90-directed proteostasis in mitochondria regulates tumour cell metabolism, and may provide a tractable target for cancer therapy. Reprogramming of tumour cell metabolism [1] is increasingly recognized as a multifaceted disease driver, enhancing biomass expansion [2] , and promoting various mechanisms of oncogenic signalling [3] . Although these processes have been mostly studied in the context of aerobic glycolysis, the so-called Warburg effect [3] , there is evidence that mitochondria continue to have an important role in tumour metabolism [4] , [5] , and organelle-driven oxidative phosphorylation has been associated with tumorigenic potential [6] , drug resistance [7] , [8] and enhanced tumour cell survival [9] . Harnessing these pathways may open new prospects for cancer therapy [10] , but the regulators of mitochondrial homeostasis in tumours have remained largely elusive, and their potential suitability as drug candidates is unknown. With a complex, multi-compartment topology, dependence on import of nuclear-encoded proteins and production of protein-modifying reactive oxygen species (ROS), mitochondria must tightly control their protein folding environment [11] . This is indispensable to maintain metabolic output [2] , ensure organelle integrity [12] and prevent the consequences of an unfolded protein response, which may result in cell death [13] . Buffering mitochondrial proteotoxic stress, especially in the protein-dense and energy-producing organelle matrix [14] , relies on adaptive responses mediated by molecular chaperones and AAA proteases [15] , and dysregulation of these mechanisms has been linked to human diseases, including neurodegeneration and cancer [14] . In this context, a pool of ATPase-directed molecular chaperones, including heat shock protein 90 (Hsp90) [16] and its related homologue, TNF receptor-associate protein-1 (TRAP-1) [17] localize to the mitochondria, almost exclusively in tumour cells [18] . The molecular requirements for the selective accumulation of these chaperones in tumour mitochondria have not been completely elucidated. However, there is evidence that both Hsp90 and TRAP-1 form overlapping complexes with mitochondrial proteins, including cyclophilin D (CypD), a component of the permeability transition pore and control their folding [19] . Accordingly, inhibition of Hsp90 and TRAP-1 chaperone activity selectively in mitochondria triggered acute organelle dysfunction [20] , defective hexokinase II (HK-II)-dependent [2] ATP production [21] , and anticancer activity in preclinical tumour models, in vivo [19] . In this study, we examined the role of Hsp90-directed mitochondrial protein folding on cellular homeostasis. Using combined proteomics and metabolomics approaches, we found that mitochondrial Hsp90 and TRAP-1 are global regulators of tumour metabolic reprogramming, including oxidative phosphorylation, and are required for disease maintenance. Identification of a mitochondrial Hsp90 proteome We began this study by setting up a preliminary proteomics screen to identify regulators of mitochondrial protein homeostasis, or proteostasis, in tumours. For these experiments, we used non-cytotoxic concentrations of Gamitrinib (GA mitochondrial matrix inhibitor), a mitochondrial-targeted, small molecule ATPase antagonist that inhibits the chaperone activity of both Hsp90 and TRAP-1 in tumours [20] . Treatment of glioblastoma LN229 cells with non-cytotoxic concentrations of Gamitrinib [21] caused the accumulation of aggregated and misfolded proteins, characterized by resistance to detergent solubilization ( Supplementary Fig. S1 ). Preliminary mass spectrometry analysis of selected bands showing higher intensities with Gamitrinib treatment identified 96 mitochondrial proteins ( Supplementary Data 1 ). Forty-four of these proteins based on spectral counts were elevated by more than threefold after Gamitrinib treatment, indicating a requirement of Hsp90 for their folding. Although gel-based comparison ( Supplementary Fig. S1 ) provides high detection sensitivity for specific bands, individual bands are not single proteins, and slight differences in band excision between control and Gamitrinib treatment can produce artificial differences. To minimize this concern, this experiment focused primarily on band differences at the 2% CHAPS condition, where protein complexity was the lowest, but not necessarily where the largest fold change occurred. To independently validate these initial results, we next performed unbiased proteomics studies using stable isotope labelling by amino acids in culture (SILAC) of control or Gamitrinib-treated cells. Of the original 44 proteins of the mitochondrial Hsp90 proteome identified by 1D mass spectrometry, 33 were independently confirmed for response to Gamitrinib in SILAC experiments ( Fig. 1a ). Of the remaining 11 proteins, 7 were below adequate detection levels for SILAC quantification, and 4 did not show significant changes. 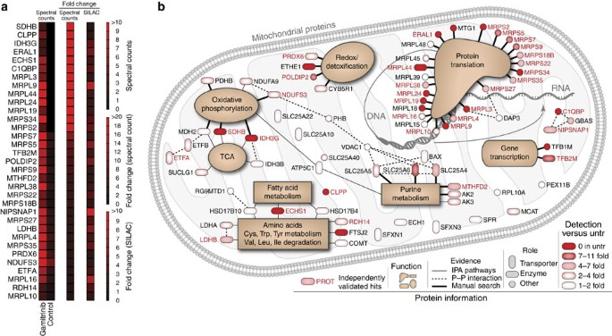Figure 1: Mitochondrial Hsp90 proteome. (a) LN229 cells were treated with vehicle (Control) or non-cytotoxic concentrations of mitochondrial-targeted Hsp90 inhibitor, Gamitrinib, and detergent-insoluble mitochondrial proteins were identified by one dimensional mass spectrometry (spectral counts), or, alternatively, by SILAC technology. The heat map quantifies changes in protein solubility (>3-fold cutoff) between the treatments assessed using the two independent proteomics approaches. (b) Schematic representation of the mitochondrial Hsp90 proteome. Proteins are annotated with functions based on literature search and information from Ingenuity software, which was also used to determine known direct protein–protein interactions. All proteins are colour coded to reflect the magnitude of difference in detection between treated and untreated (untr) samples. Proteins marked in ‘red’ exhibited a >3-fold change difference after Gamitrinib treatment compared with control, and were independently confirmed by both one dimensional mass spectrometry and SILAC technology. Figure 1: Mitochondrial Hsp90 proteome. ( a ) LN229 cells were treated with vehicle (Control) or non-cytotoxic concentrations of mitochondrial-targeted Hsp90 inhibitor, Gamitrinib, and detergent-insoluble mitochondrial proteins were identified by one dimensional mass spectrometry (spectral counts), or, alternatively, by SILAC technology. The heat map quantifies changes in protein solubility (>3-fold cutoff) between the treatments assessed using the two independent proteomics approaches. ( b ) Schematic representation of the mitochondrial Hsp90 proteome. Proteins are annotated with functions based on literature search and information from Ingenuity software, which was also used to determine known direct protein–protein interactions. All proteins are colour coded to reflect the magnitude of difference in detection between treated and untreated (untr) samples. Proteins marked in ‘red’ exhibited a >3-fold change difference after Gamitrinib treatment compared with control, and were independently confirmed by both one dimensional mass spectrometry and SILAC technology. Full size image These verified mitochondrial Hsp90-regulated proteins ( Fig. 1a and Supplementary Table S1 ) comprised the following: transcription factors TFB1M and TFB2M involved in organelle gene expression [22] and glucose homeostasis [23] ; ribosomal proteins ( MRPLs, MTG1 and ERAL1 ) associated with RNA translation [24] , [25] , [26] ; regulators of purine biosynthesis and the methyl cycle ( MTHFD2 ) [27] ; and effectors of oxidative phosphorylation [2] , including SDHB , IDH3G, NDUFS3 , PDHB and MDH2 (ref. 28 ) ( Fig. 1b ). Mitochondrial proteins participating in redox status and detoxification pathways ( PRDX6, POLDIP2, CYB5R1 and ETHE1 ) [29] , [30] , [31] were also identified in the mitochondrial Hsp90 proteome ( Fig. 1b ). Mitochondrial Hsp90 regulation of tumour metabolism The impact of a mitochondrial Hsp90 proteome ( Fig. 1b ) on cellular homeostasis was next investigated. For these experiments, we quantified the level of 301 individual metabolites in prostate adenocarcinoma PC3 cells treated with non-cytotoxic concentrations of Gamitrinib [21] or, alternatively, silenced for expression of TRAP-1 by small interfering RNA (siRNA) [21] . Both approaches produced global defects in tumour cell metabolism ( Supplementary Data 2 ). Consistent with a requirement of Hsp90 for oxidative phosphorylation ( Fig. 1b ), Gamitrinib-treated cells exhibited aberrant accumulation of citric acid cycle metabolites, succinate, fumarate and malate ( Fig. 2a ). This was associated with altered glutaminolysis (elevation in glutamine and α-ketoglutarate) ( Supplementary Fig. S2 ) and deregulated fatty acid metabolism ( Fig. 2b ), leading to higher levels of palmitate and linoleate, increased long chain fatty acid transport into mitochondria (elevation of palmitoylcarnitine and stearoylcarnitine), and excess lipid oxidation (accumulation of the ketone body 3-hydroxybutyrate ( Supplementary Fig. S3 ). Mitochondrial Hsp90-targeted cells also showed increased AMP/ATP ratio ( Supplementary Fig. S3 ), indicative of cellular starvation, and consistent with the loss of ATP production, phosphorylation of the energy sensor, AMP-activated kinase (AMPK), and inhibition of mammalian target of Rapamycin complex (mTORC1) observed in response to Gamitrinib [21] . 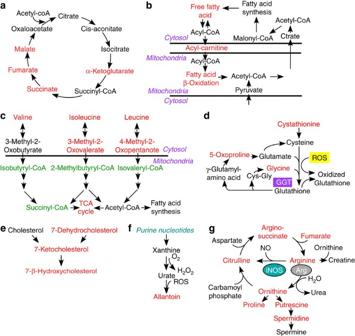Figure 2: Mitochondrial Hsp90 control of tumour cell metabolism. PC3 cells were transfected with control non-targeting siRNA or TRAP-1-directed siRNA, or, alternatively, treated with non-cytotoxic concentrations of 17-AAG (5 μM) or Gamitrinib (2.5–5 μM), and analysed for changes in expression of 301 individual metabolites by mass spectrometry. The complete summary of metabolic changes induced by targeting mitochondrial Hsp90s is presented inSupplementary Data 2. The experiment was carried out once with five independent replicates per condition tested. The metabolic pathways affected under these conditions are depicted as follows: (a) citric acid cycle; (b) fatty acid oxidation; (c) branched-chain amino acid catabolism; (d) redox status; (e) cholesterol metabolism; (f) purine nucleotide metabolism; and (g) arginine metabolism. Significant (P<0.05) changes in metabolite levels within each group (Ctrl versus TRAP-1 siRNA or vehicle versus Gamitrinib) are indicated in red (increase) or green (decrease) using Welch’s two-samplet-test (n=5). Figure 2: Mitochondrial Hsp90 control of tumour cell metabolism. PC3 cells were transfected with control non-targeting siRNA or TRAP-1-directed siRNA, or, alternatively, treated with non-cytotoxic concentrations of 17-AAG (5 μM) or Gamitrinib (2.5–5 μM), and analysed for changes in expression of 301 individual metabolites by mass spectrometry. The complete summary of metabolic changes induced by targeting mitochondrial Hsp90s is presented in Supplementary Data 2 . The experiment was carried out once with five independent replicates per condition tested. The metabolic pathways affected under these conditions are depicted as follows: ( a ) citric acid cycle; ( b ) fatty acid oxidation; ( c ) branched-chain amino acid catabolism; ( d ) redox status; ( e ) cholesterol metabolism; ( f ) purine nucleotide metabolism; and ( g ) arginine metabolism. Significant ( P <0.05) changes in metabolite levels within each group (Ctrl versus TRAP-1 siRNA or vehicle versus Gamitrinib) are indicated in red (increase) or green (decrease) using Welch’s two-sample t -test ( n =5). Full size image Targeting mitochondrial Hsp90s impaired the catabolism of branched-chain amino acids, with accumulation of valine, isoleucine and leucine ( Fig. 2c ), and decreased levels of branched-chain amino acid catabolites, isobutyryl-carnitine, succinylcarnitine, 2-methylbutyryl-carnitine and isovaleryl-carnitine ( Fig. 2c , Supplementary Fig. S4 ). This was associated with defects in redox status ( Fig. 2d ), cholesterol homeostasis ( Fig. 2e ) and purine nucleotide metabolism ( Fig. 2f ), resulting in higher levels of cholesterol metabolites associated with lipid peroxidation, ROS-dependent allantoin generation ( Fig. 2f , Supplementary Fig. S5 ), and increased oxidized glutathione, cysteine-glutathione disulphide and the glutathione catabolic product, 5-oxoproline ( Supplementary Fig. S6 ). Increased ROS production under these conditions may result from dysfunctional mitochondrial metabolism (see above), and/or increased nitric oxide generation from arginine, a possibility suggested by the accumulation of citrulline under these conditions ( Fig. 2g , Supplementary Fig. S7 ). Overall, Gamitrinib treatment produced more extensive changes in the tumour metabolome, compared with siRNA silencing of TRAP-1 ( Fig. 2 and Supplementary Figs S2–S7 ). This may reflect incomplete TRAP-1 knockdown by siRNA, or, alternatively, compensatory mechanisms provided by mitochondrial Hsp90, which is inhibited by Gamitrinib, but not by TRAP-1 knockdown. As a control, treatment of PC3 cells with 17-allylamino 17-demethoxygeldanamycin (17-AAG), which inhibits Hsp90 in the cytosol, but not mitochondria [20] , or transfection of a control, non-targeting siRNA, had minimal effects on metabolic pathways ( Supplementary Figs S2–7 ). In previous experiments, addition of the triphenylphosphonium ‘mitochondriotropic’ moiety, alone or in the presence of 17-AAG, had no effect on mitochondrial function [20] . Mechanism of mitochondrial Hsp90 control of tumour metabolism To elucidate how mitochondrial Hsp90s regulate tumour bioenergetics, we next focused on SDHB, the iron–sulphur subunit of ETC Complex II [32] , which required Hsp90s for proper folding ( Fig. 1a , Supplementary Tables S1, Supplementary Data 1 ), and functional activity ( Supplementary Fig. S2 ). Treatment of tumour cells with Gamitrinib caused insolubility of Complex II over a range of detergent concentrations ( Fig. 3a and Supplementary Fig. S8a ). In contrast, mitochondrial proteins comprising other ETC Complexes (I, IV, III and V) were minimally affected ( Fig. 3a ). Immune complexes precipitated from mitochondrial fractions of tumour cells with two independent antibodies to SDHB, but not control IgG, contained TRAP-1, in vivo ( Supplementary Fig. S8b ). In addition, immunoprecipitated SDHB associated with recombinant TRAP-1, in vitro ( Supplementary Fig. S8c ), demonstrating that these two proteins interact in tumour mitochondria. Suggestive of a chaperone-‘client protein’ recognition [33] , this interaction was required to preserve SDHB stability, as Gamitrinib treatment ( Fig. 3b ), or siRNA silencing of TRAP-1 ( Supplementary Fig. S8d ) caused SDHB degradation in tumour cells ( Fig. 3c ). 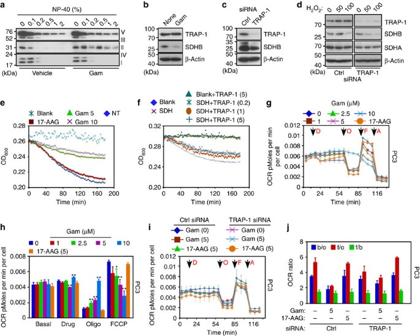Figure 3: Mitochondrial Hsp90 regulation of cellular respiration. (a) PC3 cells were treated with vehicle or Gamitrinib (Gam), solubilized in the indicated increasing concentrations of detergent (NP-40), and insoluble proteins were analysed by western blotting with an antibody cocktail to the OXPHOS complex. (b,c) PC3 cells were treated with Gamitrinib (b) or transfected with control non-targeting siRNA (Ctrl) or TRAP-1-directed siRNA (c), and analysed by western blotting. None, untreated. (d) PC3 cells were transfected as in (c), treated with the indicated increasing concentrations of H2O2(μM), and analysed by western blotting. (e) PC3 cells were treated with the indicated concentrations of Gamitrinib (Gam, μM) or 17-AAG (10 μM) and analysed for SDHB activity at the indicated time intervals. NT, not treated. (f) Endogenous Complex II (SDH) was immunoprecipitated from PC3 cells, and analysed for SDHB activity in the presence of increasing concentrations of recombinant TRAP-1 (μM). Data for panels (e,f) are from representative experiments out of at least two independent determinations. (g) PC3 cells were treated with 17-AAG (5 μM) or the indicated increasing concentrations of Gamitrinib (Gam, μM) and the OCR was measured in real time under basal condition and in response to the indicated inhibitors. Arrows indicate the time of drug addition: D, Gamitrinib (Gam) or 17-AAG; O, oligomicyin (1.25 μM); F, FCCP (0.4 μM); A, antimycin (1.8 μM). (h) The OCR was normalized by the number of cells, and the extra-mitochondrial respiration after addition of antimycin was subtracted as background. *P<0.05; **P<0.01 versus control sample at each state (two-sided unpairedt-test). (i) PC3 cells were transfected with control (Ctrl) siRNA or TRAP-1-directed siRNA, treated with Gamitrinib (Gam, μM) or 17-AAG and analysed for OCR as in (g). (j) Quantification of OCR ratio between: b/o, basal condition (before any addition) and after oligomycin addition; f/o, after FCCP and oligomycin addition; f/b, after FCCP addition and basal condition in PC3 cells transfected with control siRNA (Ctrl) or TRAP-1-directed siRNA. *P<0.05; **P<0.01 (two-sided unpairedt-test). For all OCR experiments, data are representative of two independent experiments carried out in triplicate, mean±s.d. Figure 3: Mitochondrial Hsp90 regulation of cellular respiration. ( a ) PC3 cells were treated with vehicle or Gamitrinib (Gam), solubilized in the indicated increasing concentrations of detergent (NP-40), and insoluble proteins were analysed by western blotting with an antibody cocktail to the OXPHOS complex. ( b , c ) PC3 cells were treated with Gamitrinib ( b ) or transfected with control non-targeting siRNA (Ctrl) or TRAP-1-directed siRNA ( c ), and analysed by western blotting. None, untreated. ( d ) PC3 cells were transfected as in ( c ), treated with the indicated increasing concentrations of H 2 O 2 (μM), and analysed by western blotting. ( e ) PC3 cells were treated with the indicated concentrations of Gamitrinib (Gam, μM) or 17-AAG (10 μM) and analysed for SDHB activity at the indicated time intervals. NT, not treated. ( f ) Endogenous Complex II (SDH) was immunoprecipitated from PC3 cells, and analysed for SDHB activity in the presence of increasing concentrations of recombinant TRAP-1 (μM). Data for panels ( e , f ) are from representative experiments out of at least two independent determinations. ( g ) PC3 cells were treated with 17-AAG (5 μM) or the indicated increasing concentrations of Gamitrinib (Gam, μM) and the OCR was measured in real time under basal condition and in response to the indicated inhibitors. Arrows indicate the time of drug addition: D, Gamitrinib (Gam) or 17-AAG; O, oligomicyin (1.25 μM); F, FCCP (0.4 μM); A, antimycin (1.8 μM). ( h ) The OCR was normalized by the number of cells, and the extra-mitochondrial respiration after addition of antimycin was subtracted as background. * P <0.05; ** P <0.01 versus control sample at each state (two-sided unpaired t- test). ( i ) PC3 cells were transfected with control (Ctrl) siRNA or TRAP-1-directed siRNA, treated with Gamitrinib (Gam, μM) or 17-AAG and analysed for OCR as in ( g ). ( j ) Quantification of OCR ratio between: b/o, basal condition (before any addition) and after oligomycin addition; f/o, after FCCP and oligomycin addition; f/b, after FCCP addition and basal condition in PC3 cells transfected with control siRNA (Ctrl) or TRAP-1-directed siRNA. * P <0.05; ** P <0.01 (two-sided unpaired t- test). For all OCR experiments, data are representative of two independent experiments carried out in triplicate, mean±s.d. Full size image We next asked whether a TRAP-1–SDHB complex was important during cellular stress. In control experiments, exposure of tumour cells to concentrations >50 μM of the oxidative agent, hydrogen peroxide (H 2 O 2 ), reduced SDHB levels ( Fig. 3d ). siRNA silencing of TRAP-1 exacerbated this response and induced nearly complete loss of SDHB expression at lower H 2 O 2 concentrations ( Fig. 3d ). As a control, the expression of the flavoprotein subunit of Complex II, SDHA [28] , was not affected ( Fig. 3d ). Functionally, treatment of tumour cells with Gamitrinib inhibited Complex II activity in a concentration-dependent manner, whereas 17-AAG had no effect ( Fig. 3e ). Reciprocally, addition of recombinant TRAP-1 to SDHB immuno-affinity isolated from mitochondrial extracts enhanced Complex II activity in a concentration-dependent manner, in vitro ( Fig. 3f ). Mitochondrial Hsp90 regulation of bioenergetics stress The results above have suggested that Hsp90-directed protein folding preserves the stability and function of SDHB in tumour cells. To determine whether this mechanism regulates oxidative phosphorylation, we next quantified the respiration rates of tumour cells in real time. At the same concentrations that induce SDHB misfolding ( Fig. 3a ), and impaired mitochondrial metabolism ( Figs 1 , 2 ), Gamitrinib inhibited the oxygen consumption rate (OCR) in prostate PC3 cancer ( Fig. 3g , Supplementary Fig. S9a ), or glioblastoma LN229 ( Supplementary Fig. S9b–d ) cells, in a concentration-dependent manner. 17-AAG had no effect on OCR ( Fig. 3g , Supplementary Fig. 9 ). siRNA knockdown of TRAP-1 in PC3 ( Fig. 3i , Supplementary Fig. S10a ), or LN229 ( Supplementary Fig. S10b–d ) cells, partially attenuated the inhibition of OCR mediated by Gamitrinib, compared with control transfectants. In contrast, transfection of tumour cells with non-targeting siRNA had no effect on OCR, with or without Gamitrinib ( Fig. 3i , Supplementary Fig. S10a–d ). The partial reduction in the respiratory capacity and SDHB inhibition produced by Gamitrinib when added after siRNA silencing of TRAP-1, as compared with the near complete inhibition observed when Gamitrinib is added without prior siRNA to TRAP-1, may reflect a compensatory protective response by the mitochondria as a result of the extended partial TRAP-1 inhibition produced by siRNA knockdown of TRAP-1, potentially involving organelle Hsp90. Most tumours undergo metabolic reprogramming, and utilize aerobic glycolysis as their main energy source [3] . Therefore, we asked whether oxidative phosphorylation enabled by Hsp90-directed protein folding was important for tumour maintenance. Tumour cells transfected with control siRNA and maintained in abundant nutrients (10 mM glucose) exhibited normal cellular respiration ( Fig. 4a , Supplementary Fig. S10e ). This response was increased at lower glucose concentrations (1 mM), suggestive of a compensatory mechanism that elevates ATP output by oxidative phosphorylation during nutrient deprivation ( Fig. 4a , Supplementary Fig. S10e ). Under these experimental conditions, siRNA knockdown of TRAP-1 abolished the compensatory increase in OCR at limiting glucose concentrations (1 mM), whereas cellular respiration in 10 mM glucose was minimally affected ( Fig. 4a , Supplementary Fig. S10e ). 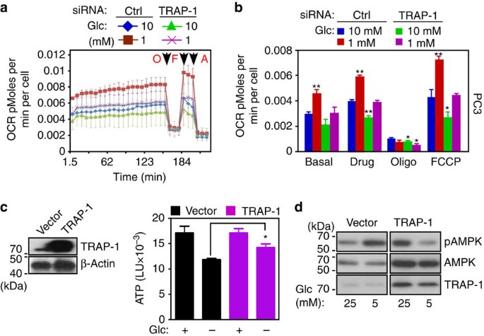Figure 4: Mitochondrial Hsp90 regulation of stress bioenergetics. (a) PC3 cells were transfected with control, non-targeting siRNA (Ctrl) or TRAP-1-directed siRNA and maintained in 1 or 10 mM glucose (Glc) for 3 h before analysis of OCR. Arrows indicate the time of drug addition: O, oligomicyin (1.25 μM); F, FCCP (0.4 μM); A, antimycin (1.8 μM). (b) OCR inawas quantified in siRNA-transfected cells in different glucose (Glc) concentrations. Data for panels (a,b) data are representative of two independent experiments carried out in triplicate, mean±s.d. *P<0.05; **P<0.01 versus control sample at each state (two-sided unpairedt-test). (c) Normal NIH3T3 fibroblasts were transfected with control vector or TRAP-1 cDNA and analysed by western blotting (left) or ATP production in the presence (+) or absence (−) of glucose (Glc, 25 mM) (right). *P=0.03 (two-sided unpairedt-test). (d) NIH3T3 fibroblasts were transfected as in (c), incubated with the indicated concentrations of glucose (Glc, mM), and analysed by western blotting. p, phosphorylated. Figure 4: Mitochondrial Hsp90 regulation of stress bioenergetics. ( a ) PC3 cells were transfected with control, non-targeting siRNA (Ctrl) or TRAP-1-directed siRNA and maintained in 1 or 10 mM glucose (Glc) for 3 h before analysis of OCR. Arrows indicate the time of drug addition: O, oligomicyin (1.25 μM); F, FCCP (0.4 μM); A, antimycin (1.8 μM). ( b ) OCR in a was quantified in siRNA-transfected cells in different glucose (Glc) concentrations. Data for panels ( a , b ) data are representative of two independent experiments carried out in triplicate, mean±s.d. * P <0.05; ** P <0.01 versus control sample at each state (two-sided unpaired t- test). ( c ) Normal NIH3T3 fibroblasts were transfected with control vector or TRAP-1 cDNA and analysed by western blotting (left) or ATP production in the presence (+) or absence (−) of glucose (Glc, 25 mM) ( right ). * P =0.03 (two-sided unpaired t -test). ( d ) NIH3T3 fibroblasts were transfected as in ( c ), incubated with the indicated concentrations of glucose (Glc, mM), and analysed by western blotting. p, phosphorylated. Full size image In reciprocal experiments, we transfected a control plasmid or TRAP-1 cDNA in normal NIH3T3 fibroblasts ( Fig. 4c ), which have low endogenous levels of mitochondrial Hsp90 and TRAP-1 (ref. 18 ). NIH3T3 fibroblasts transfected with control cDNA exhibited reduced ATP production ( Fig. 4c ), and phosphorylation of AMPK ( Fig. 4d ) at limiting glucose concentrations, consistent with cellular starvation. In contrast, transfection of TRAP-1 restored ATP production ( Fig. 4c ), and reduced AMPK phosphorylation ( Fig. 4d ) at low glucose concentrations. Role of mitochondrial Hsp90s in SDH-mutant tumours These experiments suggest that Hsp90 and TRAP-1 control multiple mitochondrial pathways of bioenergetics, and their role in oxidative phosphorylation may support energy production under conditions of nutrient deprivation. To test the implications of this model for tumour cell survival, we next targeted ETC Complex II function using pharmacological inhibitors. Treatment of tumour cells with the Complex II inhibitor, thenoyltrifluoroacetone (TTFA), but not 3-nitropropionic acid, increased the expression of hypoxia-inducible factor-1α (HIF-1α) ( Fig. 5a ), an oncogenic transcription factor implicated in adaptive responses to cellular stress [34] . Inhibition of mitochondrial Hsp90s with Gamitrinib ( Fig. 5b ), or siRNA silencing of TRAP-1 ( Fig. 5c ), was insufficient, alone, to modulate HIF-1α levels, whereas both treatments strongly enhanced TTFA induction of HIF-1α in tumour cells ( Fig. 5b ). In parallel experiments, tumour cells exposed to hypoxia exhibited increased recruitment of Hsp90 to mitochondria, compared with cytosol ( Fig. 5d ), and this response was reversed by HIF-1α silencing by siRNA ( Fig. 5f ). The mitochondrial pool of HK-II was also increased under hypoxic conditions ( Fig. 5d ), and this response was also abolished by siRNA knockdown of HIF-1α ( Fig. 5f ). In contrast, normoxic conditions ( Fig. 5d ), or transfection of tumour cells with non-targeting siRNA ( Fig. 5f ) had no effect. 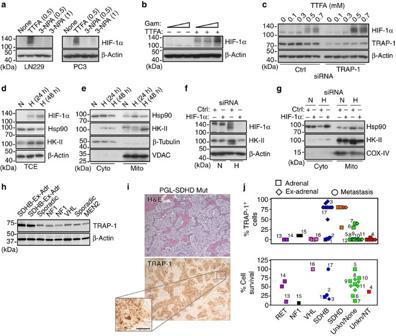Figure 5: TRAP-1–SDHB complex regulates HIF-1α-directed tumorigenesis. (a) The indicated tumour cell types (LN229 or PC3 cells) were treated with the various concentrations (mM) of the SDHB inhibitors, TTFA or 3-nitropropionic acid (3-NPA) and analysed by western blotting. (b) PC3 cells were treated with increasing concentrations of Gamitrinib (Gam, 0, 2.5, 5 μM) in the absence (−) or presence (+) of TTFA (0.3 mM) and analysed by western blotting. (c) LN229 cells were transfected with control siRNA (Ctrl) or TRAP-1-directed siRNA and analysed by western blotting in the presence of the indicated increasing concentrations of TTFA. (d,e) PC3 cells were maintained under conditions of hypoxia (H, 0.5% O2, 5% CO2, and 94% N2for 24 h) or normoxia (N), and analysed by western blotting in total cell extracts (TCE) (d), or fractionated cytosolic (Cyto) or mitochondrial (Mito) extracts (e). VDAC or β-tubulin was used as a mitochondrial or cytosolic marker, respectively. (f) PC3 cells were transfected with control siRNA (Ctrl) or HIF-1α-directed siRNA, maintained in normoxia (N) or hypoxia (H) conditions, and analysed by western blotting. (g) PC3 cells were transfected and treated as in (f), and isolated cytosolic (Cyto) or mitochondrial (Mito) fractions were analysed by western blotting. COX-IV was used as a mitochondrial marker. (h) Patient-derived tissue samples of PCC/PGL were analysed by western blotting. The mutational status of each tumour is indicated. Ex-Adr, extra-adrenal localization. (i) A tissue sample of extra-adrenal PGL withSDHDmutation, showing a typical nest-like (‘Zellballen’) growth pattern was stained with hematoxylin/eosin (H&E, top) or TRAP-1 (bottom), by immunohistochemistry. Scale bar, 50 μm. (j) Quantification of immunohistochemical expression of TRAP-1 in PCC/PGL cases with the indicated mutational status (top). Cells from the various tumour samples were maintained in culture and analysed for killing by Gamitrinib (10 μM for 2 weeks) (bottom) measured by counts of tyrosine hydroxylase-positive cells counted in an area defined by a randomly placed 22 × 22 mm2coverslips in 35 mm round culture dishes. Each point represents a single tumour. Paired samples of the same tumour were available in 12 instances and are indicated by matching numbers. Data are from a representative experiment. Figure 5: TRAP-1–SDHB complex regulates HIF-1α-directed tumorigenesis. ( a ) The indicated tumour cell types (LN229 or PC3 cells) were treated with the various concentrations (mM) of the SDHB inhibitors, TTFA or 3-nitropropionic acid (3-NPA) and analysed by western blotting. ( b ) PC3 cells were treated with increasing concentrations of Gamitrinib (Gam, 0, 2.5, 5 μM) in the absence (−) or presence (+) of TTFA (0.3 mM) and analysed by western blotting. ( c ) LN229 cells were transfected with control siRNA (Ctrl) or TRAP-1-directed siRNA and analysed by western blotting in the presence of the indicated increasing concentrations of TTFA. ( d , e ) PC3 cells were maintained under conditions of hypoxia (H, 0.5% O 2 , 5% CO 2 , and 94% N 2 for 24 h) or normoxia (N), and analysed by western blotting in total cell extracts (TCE) ( d ), or fractionated cytosolic (Cyto) or mitochondrial (Mito) extracts ( e ). VDAC or β-tubulin was used as a mitochondrial or cytosolic marker, respectively. ( f ) PC3 cells were transfected with control siRNA (Ctrl) or HIF-1α-directed siRNA, maintained in normoxia (N) or hypoxia (H) conditions, and analysed by western blotting. ( g ) PC3 cells were transfected and treated as in ( f ), and isolated cytosolic (Cyto) or mitochondrial (Mito) fractions were analysed by western blotting. COX-IV was used as a mitochondrial marker. ( h ) Patient-derived tissue samples of PCC/PGL were analysed by western blotting. The mutational status of each tumour is indicated. Ex-Adr, extra-adrenal localization. ( i ) A tissue sample of extra-adrenal PGL with SDHD mutation, showing a typical nest-like (‘Zellballen’) growth pattern was stained with hematoxylin/eosin (H&E, top) or TRAP-1 (bottom), by immunohistochemistry. Scale bar, 50 μm. ( j ) Quantification of immunohistochemical expression of TRAP-1 in PCC/PGL cases with the indicated mutational status (top). Cells from the various tumour samples were maintained in culture and analysed for killing by Gamitrinib (10 μM for 2 weeks) (bottom) measured by counts of tyrosine hydroxylase-positive cells counted in an area defined by a randomly placed 22 × 22 mm 2 coverslips in 35 mm round culture dishes. Each point represents a single tumour. Paired samples of the same tumour were available in 12 instances and are indicated by matching numbers. Data are from a representative experiment. Full size image Mutations in Complex II [35] , including SDHB [36] , have been linked to hereditary or sporadic pheochromocytoma (PCC) [37] , and paraganglioma (PGL) [38] , potentially through a mechanism of HIF-1α-dependent tumorigenesis [39] . Consistent with HIF-1α-dependent accumulation of Hsp90 to mitochondria after Complex II inhibition ( Fig. 5e ), TRAP-1 was strongly expressed in PCC/PGL samples carrying SDHB and SDHD mutations, compared with tumours with mutations in RET , NF1 and VHL , or of unknown genotype ( Fig. 5h ). Functionally, PCC/PGL tumours with Complex II mutations and high levels of TRAP-1 ( Fig. 5j ) were more sensitive to Gamitrinib-mediated killing, in vitro ( Fig. 5j ), suggesting a compensatory pro-survival role of mitochondrial Hsp90s in transformed cells with defective oxidative phosphorylation [39] . In this study, we have identified mitochondrial Hsp90s [18] as global regulators of tumour cell metabolism, including oxidative phosphorylation and redox networks. This pathway hinges on chaperone-directed protein folding in mitochondria [15] , and affects a discrete Hsp90/TRAP-1 [18] proteome intercalated in multiple, fundamental pathways of cellular homeostasis. This mechanism may be ideally suited to buffer the risk of proteotoxic stress in transformed cells with high biosynthetic needs [19] , preserve organelle integrity against CypD-dependent apoptosis [20] and maintain multiple sources of energy production, including HK-II-dependent glycolysis [21] , and oxidative phosphorylation (this study), especially under stress conditions of hypoxia and nutrient deprivation. The considerable interest in aerobic glycolysis [3] as a central feature of tumour metabolic reprogramming [1] , together with the signalling role of oncogenes in these responses [40] , have brought into question the function of mitochondrial bioenergetics, and in particular oxidative phosphorylation, in tumour maintenance [28] . However, recent studies have suggested that mitochondrial oxidative phosphorylation continues to remain critical for tumour cells [6] , favouring resistance to therapy [7] , [8] and promoting cell survival [9] . The data presented here provide a mechanistic framework in support of these observations, and identify Hsp90/TRAP-1-directed protein folding in mitochondria [18] as a key requirement of oxidative phosphorylation in tumours. This involved the formation of physical complex(es) between Hsp90/TRAP-1 and the iron–sulphur subunit of mitochondrial ETC Complex II, SDHB [32] , preserving its folding, stability and enzymatic function under oxidative stress. Functionally, Hsp90/TRAP-1 regulation of SDHB maintained energy production under conditions of low nutrients and hypoxia, which are hallmarks of tumour growth, in vivo [41] , and dampened biochemical signals of cellular starvation that are typically associated with tumour suppression [42] . SDHB [32] has attracted attention as a gene mutated in certain human neuroendocrine tumours [36] . The molecular requirements of how these mutations contribute to malignancy are still being worked out [36] , but one consequence of pharmacological or genetic inactivation of SDHB observed here was an increased recruitment of Hsp90 to mitochondria [18] . This pathway required HIF-1α, which is deregulated in SDHB-mutant tumours, and may potentially contribute to disease maintenance [39] . The increased accumulation of mitochondrial Hsp90s under these conditions may help compensate for the impaired oxidative phosphorylation resulting from defective SDHB function [36] , enhancing organelle integrity against CypD-mediated permeability transition [18] and energy production via HK-II-directed glycolysis [21] . Consistent with this model, SDHB-mutant tumour cells were more sensitive to Gamitrinib-mediated killing than other neuroendocrine malignancies, suggesting that Hsp90-directed protein folding in mitochondria provides an adaptive and potentially ‘addictive’ survival factor for these cells. There is now intense interest in pursuing aberrant tumour cell metabolism for cancer therapeutics [10] . However, inhibitors that can safely target these pathways in tumours, as opposed to normal tissues, especially with respect to oxidative phosphorylation [7] , [8] , have not been clearly identified [43] . As a mitochondrial-directed Hsp90 inhibitor [20] , Gamitrinib may be ideally suited to function as a general antagonist of tumour cell metabolism. Supported by the differential targeting of tumour, as opposed to normal mitochondria [18] , and a favourable safety profile in preclinical models [20] , Gamitrinib inhibition of mitochondrial Hsp90s may simultaneously disable metabolic and survival adaptive networks in genetically heterogeneous tumours. Antibodies and reagents The following antibodies to succinate dehydrogenase complex subunit B (SDHB, 1:500, Abcam), succinate dehydrogenase complex subunit A (SDHA, 1:3000, Abcam), HK-II (1:1000, Cell Signaling), Cox-IV (1:1000, Cell Signaling), hypoxia-inducible factor-1α (HIF-1α, 1:500, Cell Signaling), Hsp90 (1:1000, BD Biosciences), Thr172-phosphorylated AMPKα (1:1000, Cell Signaling), AMPKα (1:1000, Cell Signaling), TRAP-1 (1:1000, BD Biosciences), and β-actin (1:5000, Sigma-Aldrich) were used. A total oxidative phosphorylation antibody cocktail (1:500, Mitoscience) directed against the 20-kDa subunit of Complex I (20 kDa), cytochrome C oxidase subunit II of Complex IV (22 kDa), SDHB subunit of Complex II (30 kDa), core 2 of Complex III (~50 kDa) and F1α (ATP synthase) of Complex V (~60 kDa) was used. The complete chemical synthesis, HPLC profile, and mass spectrometry of mitochondrial-targeted small molecule Hsp90 antagonist, Gamitrinib has been reported [20] . The Gamitrinib variant containing triphenylphosphonium as a mitochondrial-targeting moiety [20] was used in this study. Non-mitochondrially directed Hsp90 inhibitor, 17-AAG was obtained from LC-Laboratories. Oligomycin, carbonyl cyanide p-trifluoromethoxyphenylhydrazone (FCCP), antimycin A, 3-nitropropionic acid and (TTFA) were obtained from Sigma-Aldrich. Transfections For gene knockdown experiments, tumour cells were transfected using control, non-targeting siRNA pool (Dharmacon, cat. no. D-001810) or specific ON-Target SMARTpool siRNAs to TRAP-1 (Dharmacon, cat. no. L-010104) or HIF-1α (Dharmacon, cat. no. L-004018). The various siRNAs were transfected at 10–30 nM using Oligofectamine (Invitrogen). Transfection of plasmid DNA was carried out with Lipofectamine (Invitrogen), as described [20] . Subcellular fractionation Mitochondrial fractions were isolated from Gamitrinib-treated LN229 cells (0–20 μM for 5 h) using an ApoAlert cell fractionation kit (Clontech), as described [20] . Briefly, LN229 cells or PC3 cells were mechanically disrupted by 70 strokes with a Dounce homogenizer in isolation buffer containing 1 mM DTT plus protease inhibitor cocktail. Cell debris was removed by centrifugation at 700 g for 10 min. The supernatant was further centrifuged at 10,000 g for 25 min, and supernatants or mitochondrial pellets were processed for further analysis. Mitochondrial protein folding Mitochondrial fractions were isolated from vehicle- or Gamitrinib-treated LN229 cells (5 μM for 12 h), and suspended in equal volume of mitochondrial fractionation buffer containing increasing concentrations of CHAPS (0, 0.05, 0.1, 0.2, 0.5, 1 or 2%). Samples were incubated for 20 min on ice and detergent-insoluble protein aggregates were recovered by centrifugation (20,000 g ) for 20 min. Pelleted proteins were separated by SDS-gel electrophoresis and visualized by silver staining (Sigma-Aldrich). Proteomics studies To identify mitochondrial proteins that require organelle Hsp90s for proper folding and/or activity (mitochondrial Hsp90 proteome), individual silver-stained bands isolated from mitochondrial fractions of vehicle or Gamitrinib-treated LN229 cells were analysed by 1D MS (see Supplementary Methods ). As an independent experimental approach, global proteomics analysis of vehicle or Gamitrinib-treated LN229 cells was carried out by SILAC technology (see Supplementary Methods ). Changes in the expression of 301 metabolites were determined by ultrahigh performance liquid chromatography/mass spectroscopy and gas chromatography/mass spectroscopy in PC3 cells treated with vehicle or Gamitrinib (2.5, 5 μM), non-mitochondrial-targeted 17-AAG (5 μM), or alternatively, transfected with control non-targeting or TRAP-1-directed siRNA (see Supplementary Methods ). Purification of TRAP-1 proteins NIH3T3 cells were transfected with human TRAP-1-Myc plasmid cDNA. After 48 h, cells were washed with PBS and lysed in PBS containing 1% TX-100 plus phosphatase inhibitor cocktail (Roche). Lysates were centrifuged at 14,000 g for 10 min at 4 °C, and c-Myc-tagged TRAP-1 proteins were isolated by immunoprecipitation with an antibody to c-Myc coupled to agarose beads (Sigma-Aldrich). Samples were then washed five times with lysis buffer, and TRAP-1-myc was eluted from the immune complex with 100 μg ml −1 c-Myc peptide (Sigma-Aldrich) in PBS. To eliminate free c-Myc peptide and further enrich eluted TRAP-1-containing material, samples were purified with centrifugal filter (30 K, Millipore). SDH activity assay Tumour cells were analysed for SDH complex activity as reduction of the dye 2,6-dichlorophenolindophenol, which recycles the substrate ubiquinone using Complex II enzyme activity. Briefly, mitochondria isolated from PC3 or LN229 cells were lysed in enzyme assay buffer containing 1% N -dodecyl-β- D -maltopyranoside plus protease inhibitors (Roche) for 1 h at 4 °C under constant agitation. After centrifugation at 15,000 g for 20 min at 4 °C, supernatants were loaded on anti-Complex II antibody-coated 96-well plates, and incubated with increasing concentrations of recombinant TRAP-1 for 2 h. Enzyme activity was determined from SDH-dependent reduction of dye 2,6-dichlorophenolindophenol, and quantified as changes in absorbance at 600 nm for 3 h at 2 min intervals using a plate reader (Beckman Coulter). Cellular respiration OCRs were assayed using the Extracellular Flux System 24 Instrument (Seahorse Bioscience, Billerica, MD). PC3 or LN229 cells were grown in standard media and after trypsinization and re-suspension in growth media, 25,000 cells were plated in each well of a Seahorse XF24 cell culture plate (100 μl volume). After 4-h incubation to allow the cells to adhere to the plate, an additional 150 μl of media was added to each well, and the cells were grown for 24 h at 37 °C with 5% CO 2 . The media was then exchanged with unbuffered DMEM XF assay media (Seahorse Bioscience) supplemented with 2 mM glutaMAX, 1 mM sodium pyruvate and 5 mM glucose (pH 7.4 at 37 °C), and equilibrated for 30 min at 37 °C and ~0.04% CO 2 before the experiment. Cellular oxygen consumption was monitored in basal condition (before any addition) and after addition of oligomycin (1.25 μM), FCCP (0.4 μM) and antimycin (1.8 μM), all dissolved in DMSO. The three drugs were injected into the XF24 sequentially, and the OCRs measured using the extracellular flux analyser with three cycles of mixing (150 s), waiting (120 s) and measuring (210 s). This cycle was repeated following each injection [44] . To test the effect of mitochondrial Hsp90s on cellular respiration, PC3 or LN229 cells were treated with non-cytotoxic concentrations of Gamitrinib (0–10 μM) or 17-AAG (2.5–5 μM) and continuously analysed for OCR changes. Alternatively, cells were transfected with control or TRAP-1-directed siRNA and analysed after 24–36 h. Patient samples All experiments involving patient-derived material were approved by the Tufts Medical Center Institutional Review Board following informed consent. A series of genetically characterized PCC/PGL with documented mutations of major susceptibility genes ( n =10, SDHB ; 6 SDHD ; 4 VHL; 3 RET ; 2 NF1 ), apparently sporadic PCC/PGL ( n =22) and normal human adrenal medulla was examined in this study. All of the tumours with VHL , RET or NF1 mutations were intra-adrenal, while 10/13 with SDHB, 3/6 with SDHD , and 10/25 with no known mutations were extra-adrenal. Two of the extra-adrenal tumours with SDHD mutations were in the head or neck and the remainder retroperitoneal. For four of the tumours with SDHB mutations, tissue was available only from metastatic sites. One SDHB -mutated tumour was an adrenal bed recurrence of a primary malignancy that had given rise to metastases. All of the other specimens were primary tumours. Statistical analysis Data were analysed using the two-sided unpaired t- tests using a GraphPad software package (Prism 4.0) for Windows. Data are expressed as mean±s.d. or mean±s.e.m. of multiple independent experiments. A P -value of <0.05 was considered as statistically significant. For pair-wise comparisons in metabolite screening studies, the Welch’s t-tests, Wilcoxon’s rank sum tests or ANOVA were performed. For classification studies, random forest analyses were performed. Statistical analyses are performed with the program ‘R’ http://cran.r-project.org/ . How to cite this article: Chae, Y. C. et al. Landscape of the mitochondrial Hsp90 metabolome in tumours. Nat. Commun. 4:2139 doi: 10.1038/ncomms3139 (2013).